Predicting network functions with nested patterns Identifying suitable patterns in complex biological interaction networks helps understanding network functions and allows for predictions at the pattern level: by recognizing a known pattern, one can assign its previously established function. However, current approaches fail for previously unseen patterns, when patterns overlap and when they are embedded into a new network context. Here we show how to conceptually extend pattern-based approaches. We define metabolite patterns in metabolic networks that formalize co-occurrences of metabolites. Our probabilistic framework decodes the implicit information in the networks’ metabolite patterns to predict metabolic functions. We demonstrate the predictive power by identifying ‘indicator patterns’, for instance, for enzyme classification, by predicting directions of novel reactions and of known reactions in new network contexts, and by ranking candidate network extensions for gap filling. Beyond their use in improving genome annotations and metabolic network models, we expect that the concepts transfer to other network types. To study the function of biological networks, a common reductionist approach is to identify recurring wiring patterns within a network. These network patterns are obtained by decomposing biological networks into their constituent small subnetworks ( Fig. 1 ). Network patterns that are statistically over-represented with respect to random networks of similar characteristics have been termed network motifs [1] , [2] . These motifs can act as modules that establish dynamic functions such as filters, timers or memory [1] , [2] , [3] . Correspondingly, if one detects a particular pattern that corresponds to a previously characterized network motif, one can aim to predict a function associated with this subnetwork [4] . 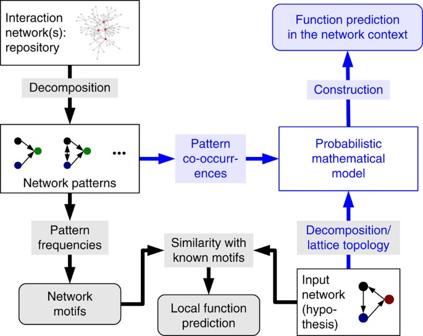Figure 1: Pattern-based prediction methods. Network motifs are obtained by decomposing larger interaction networks into patterns (subnetworks). A motif is a pattern that is over-represented compared with a random network of similar characteristics, and similarities to known network motifs have been previously used to predict local functions (black colour). Our conceptual extension (blue colour) relies on pattern co-occurrences. Biologically derived or computationally predicted (hypothetical) subnetworks are used together with the pattern statistics to construct a probabilistic mathematical model that enables function prediction in the network context. Rounded boxes denote analysis results, whereas square boxes refer to inputs and analysis steps. Figure 1: Pattern-based prediction methods. Network motifs are obtained by decomposing larger interaction networks into patterns (subnetworks). A motif is a pattern that is over-represented compared with a random network of similar characteristics, and similarities to known network motifs have been previously used to predict local functions (black colour). Our conceptual extension (blue colour) relies on pattern co-occurrences. Biologically derived or computationally predicted (hypothetical) subnetworks are used together with the pattern statistics to construct a probabilistic mathematical model that enables function prediction in the network context. Rounded boxes denote analysis results, whereas square boxes refer to inputs and analysis steps. Full size image The frequent occurrence of a pattern in a network, however, is not strictly correlated with a biological function. Network topologies reflect evolutionary origins and therefore the selection of particular functions [5] , but the specific wiring of a network may be a ‘frozen accident’ in evolution. In addition, network motifs are typically overlapping or nested—a subnetwork contains smaller patterns—such that often one cannot decide what the functionally relevant pattern is. Finally, the actual function of a given motif depends on how it is embedded into the network context. For example, the qualitative behaviour of a network motif may change dramatically depending on the inputs it receives from the rest of the network, such that the motif’s topology alone is not necessarily predictive of its biological function [6] . It is illustrative to compare this situation with the use of patterns in nucleotide sequence analysis. Nucleotide sequence motifs (short sequences with particular statistical properties) are typically employed to identify open reading frames [7] or transcription factor-binding sites [8] . In addition, limited overlaps and interactions of sequence motifs allow one to use probabilistic models to integrate information over several motifs, for instance, to quantitatively predict gene expression [9] . In contrast, the context dependence and nesting of network motifs imply largely unsolved problems for network analysis regarding (i) the identification of network patterns associated with particular functions, (ii) the inference of functions of previously unseen subnetworks ( Fig. 1 ) and (iii) the prediction of functions that are established by a pattern in a different network context, including the assessment of the hypothesis that a pattern ‘fits’ into a specific network ( Fig. 1 ). For metabolic networks, motifs have been analysed previously, suggesting that the biochemical functions are associated with particular motifs, but motif frequencies alone were not sufficient to yield high-confidence functional predictions [10] , [11] . To establish novel approaches to network analysis, however, metabolic networks are an ideal starting point. Their structure significantly constrains a metabolism’s operation in steady state, enabling the prediction of many features of its function and some of its regulation [12] , [13] . In addition, metabolic networks are well characterized, and relevant knowledge is already consistently (yet implicitly) integrated in the more than 90 available genome-scale metabolic models (GSMs) [14] . Briefly, GSMs represent the reaction structures of biochemical conversions of compounds (metabolites) along with constraints on these conversions such as those implied by directed reactions. GSMs are widely used to predict condition-dependent growth and metabolism, or to engineer metabolic pathways for various organisms [15] , [16] . However, reconstructing high-quality GSMs still requires extensive expert knowledge [17] because of erroneous and contradicting database entries [18] , [19] , unknown metabolites or reactions [20] and thermodynamically infeasible or unconstrained reactions [21] . Correspondingly, improved function predictions for metabolic networks could lead to a fully automatic model construction process [22] , and help in closing the gap between the number of sequenced genomes and reconstructed GSMs [23] . Here we demonstrate that decomposing metabolic networks as they are represented by GSMs into metabolite patterns allows us to leverage information implicitly encoded in these GSMs by deriving statistics on patterns and the association of patterns with biological functions. Our probabilistic methods explicitly incorporate information from all patterns to predict unknown reaction and network characteristics such as classes of enzymes that catalyse metabolic reactions, constraints on fluxes through metabolic reactions and missing reactions in a new network context ( Fig. 1 ). These approaches are general, with potential applications to other types of biological networks. Metabolite patterns A metabolic network is a set of interconnected biochemical reactions in which metabolites are converted into each other (see Fig. 2a for an example; formal concepts were recently reviewed [11] ). Here, we are interested in predicting properties of individual reactions embedded into a larger network. This includes the assessment of hypotheses on whether a network should be augmented by a specific reaction (see Fig. 1 ). A reaction can have various properties or features, such as its size (the number of different participating metabolites), its enzyme classification (EC) number (that characterizes the type of biochemical reaction), its intracellular localization or its direction. A metabolite pattern is a substructure of a reaction defined by a subset of metabolites for each side of the considered reaction (see Supplementary Methods for formal definitions). A metabolite pattern, hence, encodes co-occurrences of metabolites within the same reaction; its size is again the number of its different metabolites. We denote metabolite patterns by their left- and right-hand sets of metabolites separated by a comma. For instance, reaction R3 in Fig. 2a has one pattern, (B+C, D), of size three, three patterns, (B+C, ø), (B, D), (C, D), of size two, and three patterns, (B, ø), (C, ø), (ø, D), of size one ( Fig. 2b ). Note that patterns may share metabolites and that each pattern defines a hierarchy of nested sub-patterns. 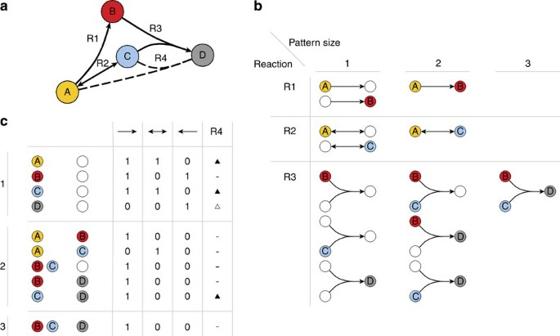Figure 2: Concept of metabolite patterns. (a) Example network of four reactions (edges R1–R4) and four metabolites (vertices A–D). Arrows show the reactions’ directions and the dashed edge represents a hypothetical reaction A+C~D (R4) with unknown direction. (b) Metabolite patterns for R1–R3 with one column per pattern size. Transparent nodes illustrate metabolites ignored by the pattern. Note that both graphs in the first column containing the C metabolite denote the same pattern (C, ø). (c) Pattern co-occurrence count-table for R1–R3 with an additional column indicating whether a pattern appears in the hypothetical reaction R4 in the corresponding (filled triangle) or in the opposite (open triangle) direction. Figure 2: Concept of metabolite patterns. ( a ) Example network of four reactions (edges R1–R4) and four metabolites (vertices A–D). Arrows show the reactions’ directions and the dashed edge represents a hypothetical reaction A+C~D (R4) with unknown direction. ( b ) Metabolite patterns for R1–R3 with one column per pattern size. Transparent nodes illustrate metabolites ignored by the pattern. Note that both graphs in the first column containing the C metabolite denote the same pattern (C, ø). ( c ) Pattern co-occurrence count-table for R1–R3 with an additional column indicating whether a pattern appears in the hypothetical reaction R4 in the corresponding (filled triangle) or in the opposite (open triangle) direction. Full size image By counting the number of occurrences of a given pattern in reactions with a particular set of features (that is, single reaction properties or combinations of reaction properties as described above), we derive a pattern count-table that represents the joint distribution of patterns and reaction features. This count-table forms the foundation for deriving pattern statistics according to the scheme in Fig. 1 to predict features of unknown reactions. Its construction is exemplified in Fig. 2c using reaction directions as the relevant reaction feature. We distinguish between unidirectional (irreversible) reactions operating in the forward (→) and backward (→) direction, and reversible (↔) reactions. For instance, R2 contributes three reversible counts to its respective patterns, and the two non-zero entries for pattern (A, ø) originate from R1 and R2. Metabolite patterns thereby provide quantifiable evidence for the relationships between (multiple) arbitrary features and reactions. For the analysis of metabolite patterns, we employed a set of experimentally validated GSMs that encode metabolic networks of various complexities and represent organisms from bacteria to humans ( Table 1 ). When we computed the basic metabolite pattern statistics—such as the distributions of pattern counts over pattern sizes—in the E. coli model iAF1260 (ref. 24) [24] as one example, we found significant occurrences of patterns larger than two. Moreover, in agreement with previous studies on motif searches in metabolic networks [25] and on general metabolic network organization [26] , the pattern frequency distribution followed a power law ( Supplementary Fig. S1 ). We therefore conclude that metabolite patterns provide relevant extensions of coupled metabolites [27] from two to arbitrary numbers of co-occurring metabolites. Table 1 GSMs used here and their key characteristics. Full size table Using patterns independently to identify reaction features Metabolite patterns are nested. For instance, the size-four pattern (ATP, ADP+H+Pi) ( Fig. 3a ) establishes a hierarchy of smaller patterns, whose counts remain constant or increase when going down this hierarchy. To identify which patterns are predictive of reaction features, however, we initially ignored pattern nesting. Reaction directions were our first feature of interest because their correct assignment is difficult and critical [17] . For GSMs, the directions are encoded by flux constraints that hold for any physiological condition. Heuristic rules that consider, for example, the production of energy equivalents are often used to assign these constraints in network reconstruction. We applied two selected heuristics [17] , [28] , [29] ( Supplementary Table S1 ) to an unconstrained E. coli iAF1260 model. In general, we defined the classification accuracy (CA) of direction assignments as consistency with manually curated GSMs. Note that this is the best available—but limited—basis for the evaluation of accuracy. The two heuristics showed an average CA of ≈43% for iAF1260 ( Supplementary Table S2 ) in contrast to an expected CA of one third for random assignments (three different reaction directions are possible). 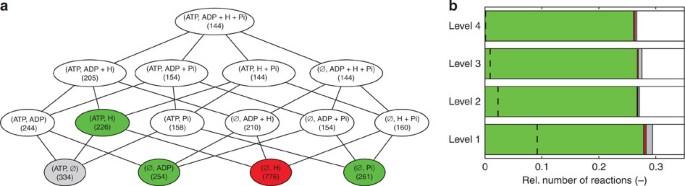Figure 3: Predictive patterns for theE. coliiAF1260 model. (a) Relationship between the most abundant patterns in theE. coliiAF1260 model, ordered by inclusion for a pattern (top) and all its sub-patterns (pattern counts in brackets). Green: indicator patterns; white: association with a direction based on indicator patterns; red: ambiguous direction; grey: not an indicator pattern because (ATP+H, ø) is ambiguous. (b) Accuracy of EC number predictions depending on EC number level (expected values indicated by dashed lines). Correct (incorrect) predictions are shown in green (red); dark (light) colours denote a reaction present in the database (only in iAF1260). Predictions that cannot be tested are shown in gray, cases where no assignment is possible in white. Figure 3: Predictive patterns for the E. coli iAF1260 model. ( a ) Relationship between the most abundant patterns in the E. coli iAF1260 model, ordered by inclusion for a pattern (top) and all its sub-patterns (pattern counts in brackets). Green: indicator patterns; white: association with a direction based on indicator patterns; red: ambiguous direction; grey: not an indicator pattern because (ATP+H, ø) is ambiguous. ( b ) Accuracy of EC number predictions depending on EC number level (expected values indicated by dashed lines). Correct (incorrect) predictions are shown in green (red); dark (light) colours denote a reaction present in the database (only in iAF1260). Predictions that cannot be tested are shown in gray, cases where no assignment is possible in white. Full size image When we computed the metabolite pattern statistics for iAF1260, we found 180 metabolite patterns that were both abundant and associated with a preferred reaction direction. Out of these 180 patterns, 51 patterns were unique for a direction and they could not be further decomposed; we call them ‘indicator patterns’ (see Supplementary Methods , Supplementary Note 1 and Supplementary Table S3 ). For instance, in the hierarchy of patterns established by (ATP, ADP+H+Pi) ( Fig. 3a ), only ADP alone uniquely determines the direction of reactions with ATP and ADP on different sides. In contrast, in reactions with pairs of redox equivalents such as (NADH, NAD), all indicator patterns have at least one additional metabolite (see Supplementary Table S4 for a summary). The indicator patterns constitute reaction rules that were derived from the entire network statistics. When we applied these inferred rules, the CA increased to ≈63% for iAF1260. For the eight GSMs marked by ‘*’ in Table 1 , the CAs were 47±7% and 50±7% for the two heuristics, and 60±9% for the indicator patterns ( Supplementary Table S2 and Supplementary Data 1 ), indicating generally improved predictions of reaction directions. Next, we focused on EC numbers, which give a hierarchical four-level description of enzyme function and categorize reactions by (bio)chemical properties. We identified weighted associations between size two patterns and EC numbers from five GSMs. We then predicted EC assignments at all four levels for the sixth model iAF1260, in which only ≈46% of the reactions have a corresponding annotation (see Supplementary Methods and Supplementary Note 2 ). An EC number could be predicted for ≈30% of all reactions with a CA of >97%, irrespective of the EC number level ( Fig. 3b ). Importantly, the transfer of EC annotations resulted in a set of 48 new predictions that can be used for improved annotation of this model, and potentially of the E. coli genome ( Supplementary Data 2 ). Relevant biochemical knowledge is thus implicitly encoded in networks and it can be leveraged already by using individual metabolite patterns independently to (re)derive relatively accurate—and intuitively comprehensible—reaction rules without exterior knowledge. Feature propagation hidden Markov model To infer functions of both previously unseen and known patterns in a new network context, we developed a constructive, probabilistic and predictive method based on hidden Markov models (HMMs) [30] . It considers all decompositions of a reaction into its metabolite patterns and computes the reaction’s feature distribution as a weighted sum of the patterns’ feature distributions. Thereby, our method leverages information from non-unique patterns, resolves conflicts between feature distributions of patterns and handles nested and overlapping patterns. Briefly, we construct a Markov chain by representing each metabolite pattern of a reaction as a vertex, as illustrated in Fig. 4 for reaction R4 (see also Fig. 2a,c ). The corresponding graph has one layer per pattern size, with the empty pattern (ø, ø) at the bottom and the entire reaction at the top. A transition from a particular pattern P1 to another pattern P2 is possible if P2 contains P1. The transition probability derives from the probability of drawing the pattern that extends P1 to P2. Hence, each path from bottom to top represents one possibility of constructing the entire reaction from patterns (see Supplementary Methods for all formal details). 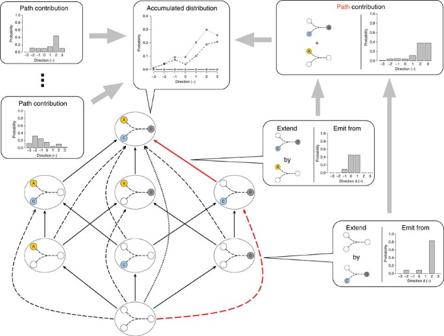Figure 4: HMM for example reaction R4: A+C~D. Each pattern corresponds to a node (ellipses), including the empty pattern (bottom node) and the full pattern (top node). Each edge has an associated extension pattern that extends a source to a target pattern, and the edge emits a direction value from a probability distribution associated to that extension pattern. Any path from bottom to top represents a unique way of composing the reaction from its patterns. For the path highlighted in red, extension patterns and emission distributions are shown. The path contributes a direction distribution to the reaction (top right box) together with its pattern composition. Accumulating evidence from all paths gives the overall direction probability distribution for the reaction in the top node (top). Accumulation of evidence after the first (full), second (dashed) and third (dotted) step of the HMM is given. A classifier compares probabilities for having a negative/zero/positive score to derive a discrete distribution. Figure 4: HMM for example reaction R4: A+C~D. Each pattern corresponds to a node (ellipses), including the empty pattern (bottom node) and the full pattern (top node). Each edge has an associated extension pattern that extends a source to a target pattern, and the edge emits a direction value from a probability distribution associated to that extension pattern. Any path from bottom to top represents a unique way of composing the reaction from its patterns. For the path highlighted in red, extension patterns and emission distributions are shown. The path contributes a direction distribution to the reaction (top right box) together with its pattern composition. Accumulating evidence from all paths gives the overall direction probability distribution for the reaction in the top node (top). Accumulation of evidence after the first (full), second (dashed) and third (dotted) step of the HMM is given. A classifier compares probabilities for having a negative/zero/positive score to derive a discrete distribution. Full size image Emissions of the HMM are modelled according to the specific feature to be predicted. For instance, for direction prediction, each transition emits a value in { +n,−n, 0} on the corresponding edge. The emission probability for each direction is derived from the direction distribution of the corresponding extension pattern associated to the edge, scaled by the size n of the extension pattern. Each possible path starting in the neutral bottom node and ending in the top node contributes to the reaction’s direction distribution in the top node (see the example path in Fig. 4 ): emitted directions are summed up to give an overall direction, weighted by the probability to choose the particular path. The reaction's feature distribution is calculated recursively by using the contributions of all possible paths. For discrete features in GSMs such as reaction directions, we compute the log-ratio score S of the probabilities of a non-positive and a non-negative direction sum and we apply classifiers on S to assign the features. For instance, S =−1.25 for R4 in Fig. 4 provides strong evidence for forward operation of the reaction (we employ the sign convention from thermodynamics where a negative formation energy corresponds to operation of a reaction in the forward direction; see Supplementary Methods for details). Prediction of reaction directions with dependent patterns To evaluate the HMM framework for reaction directions, we first performed a leave-one-out cross-validation (LOOCV) analysis by predicting the direction of each reaction using pattern statistics derived from the remaining reactions of the corresponding model. Scores for iAF1260 clearly distinguished between the original forward, reversible and backward reactions ( Supplementary Fig. S2 ). Optimized model-specific classifiers for each reaction length resulted in a CA of 78%, which is significantly higher than expected ( P =10 −4 ) when compared with randomized versions of iAF1260. We obtained similar results for the other GSMs marked by ‘*’ in Table 1 and for non-specific classifiers ( Fig. 5a ; see also Supplementary Methods and Supplementary Data 1 ), indicating robustness against model and classifier specifics. 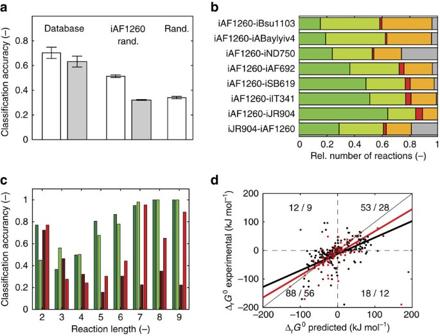Figure 5: Pattern-based prediction of reaction directions. (a) Averaged classification accuracies (mean±s.d.) for all models marked by ‘*’ inTable 1(‘database’), for random models based on iAF1260 (‘iAF1260 rand.’) and for randomly assigned reaction directions in iAF1260 (‘rand.’; see Methods). White (grey) bars indicate optimized model-specific (global) threshold parameters. (b) Inter- and intraspecies reaction direction predictions using all patterns. Colours indicate correct direction predictions (green shades), incorrect predictions (red shades), and reactions without prediction (grey). Dark shades refer to common reactions of training and target models and light shades to reactions that exist only in the target model. (c) Comparison of accuracies of pattern-based predictions (LOOCV for iAF1260, dark green; intraspecies model transfer from iJR904, light green) with those of a group contribution method36(dark red), and of previously published heuristic rules (light red) grouped by reaction length. (d) Predicted versus experimentally determined Gibbs free energy changes for IGERS37(red circles and linear regression line) and metabolite patterns (LOOCV, scaling factor 20; black). Light and dark colours for IGERS refer to reactions of high (Tanimoto coefficient T≥0.6) and low (T<0.6) similarity. Numbers show the sizes of data sets in the quadrants (dashed lines) for metabolite patterns (first entry) and IGERS (second entry). Figure 5: Pattern-based prediction of reaction directions. ( a ) Averaged classification accuracies (mean±s.d.) for all models marked by ‘*’ in Table 1 (‘database’), for random models based on iAF1260 (‘iAF1260 rand.’) and for randomly assigned reaction directions in iAF1260 (‘rand.’; see Methods). White (grey) bars indicate optimized model-specific (global) threshold parameters. ( b ) Inter- and intraspecies reaction direction predictions using all patterns. Colours indicate correct direction predictions (green shades), incorrect predictions (red shades), and reactions without prediction (grey). Dark shades refer to common reactions of training and target models and light shades to reactions that exist only in the target model. ( c ) Comparison of accuracies of pattern-based predictions (LOOCV for iAF1260, dark green; intraspecies model transfer from iJR904, light green) with those of a group contribution method [36] (dark red), and of previously published heuristic rules (light red) grouped by reaction length. ( d ) Predicted versus experimentally determined Gibbs free energy changes for IGERS [37] (red circles and linear regression line) and metabolite patterns (LOOCV, scaling factor 20; black). Light and dark colours for IGERS refer to reactions of high (Tanimoto coefficient T≥0.6) and low (T<0.6) similarity. Numbers show the sizes of data sets in the quadrants (dashed lines) for metabolite patterns (first entry) and IGERS (second entry). Full size image To transfer knowledge from existing to new models, we first predicted reaction directions for the model iAF1260 using the smaller predecessor E. coli model iJR904 (ref. 31) [31] ( Table 1 ) to derive the pattern statistics, and vice versa. With general classification parameters, our method yielded on average ≈80% correct predictions in both directions, and a majority (≈64%) of consistent assignments for reactions unique to each model ( Fig. 5b ; some directions remained undefined because iAF1260 contains additional metabolites). The more challenging prediction of metabolic functions in a different species based on pattern statistics from iAF1260 resulted in an average CA of ≈74% and coverage of ≈92% per transfer ( Fig. 5b ). Not surprisingly, we obtained the lowest accuracies for yeast, which is phylogenetically most distant from E. coli among the organisms considered. In addition, accuracies were lower for models iBsu1103 (ref. 29) [29] and iAbaylyiv4 (ref. 32) [32] that originate from different research groups and have limited similarity to the other models. Notably, when we repeated the analyses with patterns of size one only, the average CA dropped to ≈63% ( Supplementary Fig. S3 ), confirming our implicit assumption that co-occurrences of metabolites (patterns of size ≥2) carry significant information. Because the assignment of reaction directions is critical for GSM performance, we tested the models with inferred directions for functionality in terms of biomass formation, and therefore growth. Such tests can be performed by flux balance analysis (FBA) simulations, in which the model fluxes are optimized for maximal growth rate [33] . The models with inferred reaction directions showed clear growth capabilities in six out of 16 cases and for four out of eight organisms ( Supplementary Data 3 ). In particular, non-zero-predicted growth rates make these models suitable for further model optimization using established algorithms [34] ; for cases with zero growth after direction transfer, similar optimization algorithms could be developed that incorporate only a subset of the predicted direction constraints while maintaining growth. Thus, our pattern-based framework yields accurate and practically useful predictions by statistically evaluating and weighting knowledge implicitly encoded in all relevant metabolite patterns. Comparison with chemically detailed prediction methods Metabolite patterns as defined above are agnostic to the metabolites’ chemical attributes. It is therefore a priori unclear if they can yield detailed predictions on reaction chemistry or thermodynamics. Yet, the reaction direction score S can be interpreted as a quantitative approximation of the reactions’ standard Gibbs free energy changes, Δ r G ° (up to a scaling factor; see Supplementary Methods ). Because few experimental thermodynamic data are available [28] , reaction energies of chemical reactions in general are often estimated by group contribution methods that consider the additive reaction energies of chemical sub-structures [35] . Reaction directions then depend on these energies and on metabolite concentrations. For iAF1260, direction predictions based on group contribution methods [36] show an average CA of ≈36% ( Fig. 5c ). They are most accurate for short reactions, but the accuracy decreases with increasing reaction length, presumably due to error propagation when energy estimates for individual metabolites are added. Our pattern-based approach makes more accurate predictions for longer reactions because those reactions provide more patterns and pattern counts ( Fig. 5c ). Existing heuristics predict reactions with seven or more metabolites with high accuracy because the majority of those reactions (for example, ABC transporters) contains ATP as a substrate, but the heuristics do not cover all relevant metabolites, such as the redox-pairs FMN(H2) and NAD(H). However, note that a direct comparison of the results is difficult because the methods employ different prior information. We also compared our approach to the IGERS method [37] , which uses detailed chemical features to assign the experimentally determined Δ r G ° value of the most similar reaction to a reaction with unknown Δ r G °. Metabolite patterns and IGERS showed 82 and 80% prediction accuracy for the qualitative directions of 171 and 105 (out of 173 tested) reactions, respectively ( Fig. 5d , Methods and Supplementary Data 4 ). Linear correlations between quantitative predictions and experimental data were significant in both cases ( P <10 −10 ). The average correlations of IGERS were higher, but less stable under random resampling of the test data (Methods, Supplementary Fig. S4 and Supplementary Methods ). Hence, despite being agnostic about chemistry, our pattern-based approach seems largely complementary to thermodynamic and chemically detailed approaches. Gap filling Finally, we addressed pattern-based predictions in a different network context by considering the problem of gap filling, that is, the identification of missing reactions in a given metabolic network. This problem is more global than predicting reaction features, because it amounts to deciding whether a candidate reaction belongs to a specific target network, or not. Several automated gap filling methods exist [38] , but they typically require formally detectable effects of the gap [34] , additional experimental data [39] or comprehensive model annotations [40] . We aimed to rank candidate reactions according to their probability of belonging to a target GSM without computationally expensive tests of model functions or external information. For this purpose, we used a feature propagation HMM to compute a log-ratio score S that measures how closely related a candidate reaction is to the target model, compared with an average of all models in a repository. We constructed the HMM with emissions { +n,−n } for observing the reaction in the model or in our model repository, respectively. A higher score indicates that a candidate reaction more specifically belongs to the target model than to an ‘average’ metabolic model (see Supplementary Methods ). We evaluated the method by scoring 750 unique reactions across nine models for different organisms (see Table 1 for the GSMs employed, Supplementary Data 5 for the reactions considered, and Methods) to identify reactions from other models that could fill gaps in the E. coli model iAF1260. The reaction scores clearly separate by species of origin, as indicated by their cumulative probability distribution functions ( Fig. 6a ). Here, human Recon1 (ref. 41) [41] serves as a negative control and iJO1366 (ref. 42) [42] , the most recent extension of iAF1260, as a positive control. Similarly, the positions of the 10% best ranked reactions of each model ( Fig. 6b ) show a proximity of E. coli -specific reactions as well as a separation between reactions of eukaryotic (human and yeast) and prokaryotic (all other networks) origin. 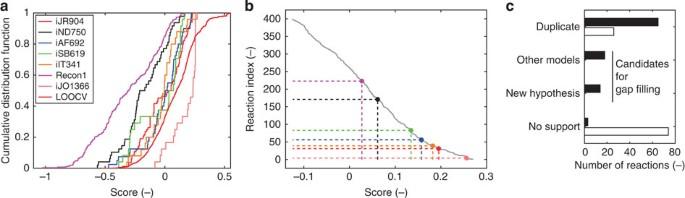Figure 6: Application of metabolite patterns to gap filling for iAF1260. (a) Cumulative probability distributions of gap filling scores after testing reactions unique to the models indicated (see alsoTable 1for model identifiers). (b) Position of top 10% reactions for unique reactions from individual models (colour coding according to (a)) in the ranked list of scores for all models; grey symbols show relations between gap filling score and rank for candidate reactions. (c) Classification of top 100 (filled bars) and bottom 100 (open bars) scored reactions according to the evidence for inclusion into iAF1260. Figure 6: Application of metabolite patterns to gap filling for iAF1260. ( a ) Cumulative probability distributions of gap filling scores after testing reactions unique to the models indicated (see also Table 1 for model identifiers). ( b ) Position of top 10% reactions for unique reactions from individual models (colour coding according to ( a )) in the ranked list of scores for all models; grey symbols show relations between gap filling score and rank for candidate reactions. ( c ) Classification of top 100 (filled bars) and bottom 100 (open bars) scored reactions according to the evidence for inclusion into iAF1260. Full size image For a more detailed analysis, we manually inspected the 100 bottom and top ranked reactions in the list of 750 candidate reactions. The bottom 100 reactions contained 26 duplicates in iAF1260 (for example, because the reaction was defined in other models without differentiating between cellular compartments), and no other candidates could be validated ( Fig. 6c ). In contrast, most of the 100 top candidates could be substantiated by further inspection. Many of these reactions were incorporated into other manually curated E. coli models and can thus be assumed correct ( Fig. 6c ). Another set of 32 reactions could be corroborated by independent evidence. Out of these 32 candidates, one reaction originated from the predecessor E. coli model iJR904, and 17 reactions originated from the successor E. coli model iJO1366. The 14 reactions shown in Table 2 constitute novel predictions, for instance, on transport mechanisms for metal ions and on the synthesis of complex lipids. Based on homology, we identified genes in E. coli that are presumably associated with those reactions ( Supplementary Table S5 and Supplementary Data 5 ), and this will allow for future experimental testing of the hypotheses. In addition, we performed functional tests of iAF1260 with and without adding the 32 candidates. In FBA simulations to determine maximal growth rates and accuracies of predictions on the viability of the organism when single genes are inactivated, the original and the extended model performed very similarly for a standard experimental data set [43] ( Supplementary Table S6 ). In addition, 29 of the 32 candidate reactions could in principle carry steady-state carry flux (see Methods) in the extended network, and the network extension rendered an additional 11 reactions in the original model functional. These tests indicate that gap filling with the candidate reactions enhances model functionality. Overall, the top 100 list was significantly enriched for E. coli -specific reactions ( P <10 −7 ) in contrast to all other organisms considered ( P >3·10 −2 ). Thus, the analysis provided strong support for the pattern-based approach to gap filling. Table 2 Candidate reactions and predicted loci for inclusion into iAF1260. Full size table Previous studies on motifs [11] and on subgraph patterns [10] demonstrated that local topologies in metabolic networks are associated with biological functions such as the localization of metabolic reactions within a cell and the non-random use of common substrates in metabolic reactions, respectively. These associations, however, were weak and not directly applicable to predict network features, also because of the focus on statistical over-representation of patterns and the restriction to patterns of a single size. Other approaches to the analysis of metabolic networks accounted for the network context in order to predict tissue-specific metabolic functions [44] , or to automatically assign genes to metabolic reactions [38] , [45] , but they require information in addition to the network topology. Similarly, existing frameworks for the automatic construction of metabolic network models involve model optimization by network-internal criteria as well as by comparison of model predictions with experimental data [46] . In contrast, our metabolite pattern-based framework relies on network topologies alone, and it predicts metabolic functions by leveraging the statistical information contained in well-curated network models. In essence, it is a constructive approach for analysing biological network features because it evaluates hypotheses by (potentially) integrating over all possible paths for constructing them, which leads to high-accuracy predictions. The predictions are complementary to those from alternative methods (such as thermodynamics or current heuristics for reaction directions), and the method allows for a systematic information transfer between different networks. In addition, we demonstrated that pattern-based methods can systematically evaluate candidate reactions with respect to their likelihood of being part of a given network (model)—which could as well be applied to computationally predicted biochemical reactions [47] . For the metabolic network application area, we therefore envisage our framework to help improve existing, and to construct new network models. More generally, the proposed framework for analysing network features using pattern statistics is generic in two regards: it could be extended to other network types, and it provides direct connections to the extensive standard theory of Markov chains and HMMs. The latter makes it easy to incorporate additional knowledge; for metabolic networks, one could consider, for example, the detailed chemical structure of metabolites, or the complicated subcellular localization of reactions in higher eukaryotes [48] . Such combined predictions would not only enable a coherent integration of existing knowledge on biological networks, but also the generation of experimentally testable hypotheses to discover new network features. Genome-scale metabolic network models We downloaded publicly available genome-scale models from the BiGG database [49] and from published Supplementary Materials . All models were translated into the BiGG naming scheme and common naming conventions [31] were used. A metabolite occurring in several compartments was associated with several distinct metabolite identifiers, and we added external reactions whenever external metabolites were either a sink or a source. Reaction constraints from the original models were used. Generation of randomized networks We consider a metabolic network with stoichiometric matrix N containing σ metabolites in r reactions. Much of our proposed method involves co-occurrences of metabolites and seeks to exploit statistically significant frequencies of such co-occurrences. Our algorithm for sampling random networks ( Supplementary Fig. S5 ) keeps all relevant statistical properties of the original network, while completely randomizing co-occurrences of metabolites. It takes the original stoichiometric matrix and repeatedly selects two reactions uniformly at random; two metabolites with the same sign of the molecularity, one in each reaction, are chosen and exchanged. Afterwards, educts and products in a reaction are repeatedly swapped. As a result, the new network has the same number of reactions and the i th reaction has the same left- and right-hand sizes as the i th original reaction. The reactions’ directions as well as their numbers of metabolites remain unchanged. Performance evaluation for reaction direction predictions To compute the statistical significance of the number of correct assignments of reaction directions, we first randomly generated 10,000 variants of each model considered by setting one half of the irreversible reactions in a model to ‘backward’ (and consequently exchanging the left- and right-hand sides of the reaction equations). For each of these models, we then computed a LOOCV of the HMM-based reaction-direction prediction. Let k be the number of these 10,000 randomly shuffled models that reach higher CA than the original model. The P -value for the CA of the original model is then given by . Assignment of EC numbers We performed EC number assignments as detailed in Supplementary Methods and evaluated the method’s performance using the iAF1260 model as test set and the remaining five BiGG models listed in Table 1 as training set. Detailed results on the identified patterns are given in Supplementary Data 2 . Specifically, we transferred the results to iAF1260 by associating all of its reactions with EC numbers. We distinguish four cases as follows: (i) an association is unique (multiple), giving exactly one (multiple) associated EC number(s); (ii) an association is either correct by containing the same EC number as the one in iAF1260, or incorrect otherwise; (iii) an association with at least one EC number is made, but its correctness cannot be established because the reaction is not annotated in iAF1260; these cases are called newly associated; (iv) finally, it is possible that no association above a given threshold is found. Note that only 957 out of 2,077 reactions in iAF1260 carry an EC number and proper evaluation is only possible on this subset. Comparison of predictors for reaction energies For detailed performance comparison, we used a previously published data set of 173 reactions [28] , for which standard Gibbs energies are available for physiological conditions. The same data set was also used as a reference set for IGERS [37] . For each reaction, we computed the reaction directionality score S , using LOOCV of the 173 reactions for calculating metabolite pattern counts. To evaluate how robust the two regressions are, we re-sampled the data by randomly selecting 1,000 sets each containing 50% of the reactions. We then calculated the linear regressions for each of these sets and evaluated the variation in the resulting coefficient r 2 . Detailed data are provided in Supplementary Data 4 . Evaluation of gap filling To evaluate the proposed method for gap filling (see Supplementary Methods ), we created a joint database using all reactions of the models iAF1260, iJR904, iIT341, iAF692, iSB619, iND750 and iJO1366 for computing the database count-table; these counts represent the ‘common biochemical reactions’. As a target model, we chose the E. coli model iAF1260. Note that this model is also a part of the joint database; its reactions are used to compute the background knowledge of biochemical reactions. We identified all reactions in the joint database that are (i) not already contained in iAF1260 and (ii) only contain metabolites also present in iAF1260. The resulting 750 reactions were then tested as candidates for gap filling in the target model and ranked according to the score computed by the HMM framework. To assess flux through novel reactions, we used the kernel matrix K (right null space) of the stoichiometric matrix N and the reaction reversibilities to determine zero-flux reactions. These reactions always have a zero rate in steady state due to the overall network structure because they are either dead-end reactions or they belong to inconsistent correlation groups [50] . Implementation and simulation All analyses and computational simulations were performed using MATLAB (The MathWorks, Natick, MA) or R ( http://www.r-project.org ). Coin-CLP ( https://projects.coin-or.org/Clp ) was used as linear programming solver for FBA. An average prediction takes ~10 min for intra- or interspecies transfer of reaction directions on a single Intel(R) Xeon(R) 2.93 GHz core. Availability The HMM-based methods are available at http://www.metanetx.org [51] ; MATLAB code is available upon request from the authors. How to cite this article : Ganter, M. et al. Predicting network functions with nested patterns. Nat. Commun. 5:3006 doi: 10.1038/ncomms4006 (2014).